Two complementary genes in a presence-absence variation contribute toindica-japonicareproductive isolation in rice Understanding the evolutionary forces in speciation is a central goal in evolutionary biology. Asian cultivated rice has two subspecies, indica and japonica , but the underlying mechanism of the partial reproductive isolation between them remains obscure. Here we show a presence-absence variation (PAV) at the Se locus functions as an indica-japonica reproductive barrier by causing hybrid sterility (HS) in indica-japonica crosses. The locus comprises two adjacent genes: ORF3 encodes a sporophytic pollen killer, whereas ORF4 protects pollen in a gametophytic manner. In F 1 of indica-japonica crosses, pollen with the japonica haplotype, which lacks the sequence containing the protective ORF4 , is aborted due to the pollen-killing effect of ORF3 from indica . Evolutionary analysis suggests ORF3 is a gene associated with the Asian cultivated rice species complex, and the PAV has contributed to the reproductive isolation between the two subspecies of Asian cultivated rice. Our analyses provide perspectives on rice inter-subspecies post-zygotic isolation, and will promote efforts to overcome reproductive barriers in indica-japonica hybrid rice breeding. Detection and characterization of structural variants (SVs) has revolutionized the understanding of the landscape of genomic and phenotypic variation in different species [1] , [2] . Presence-absence variation (PAV) is an extreme form of SV, in which a genomic segment containing one or more genes is present in some individuals but absent in others [3] . The unprecedented low cost of DNA sequencing and advances in high-quality genome assembly today make it possible to generate a wealth of data on PAVs in plant genomes [4] , [5] , [6] , [7] , [8] , [9] , [10] , [11] , [12] , [13] . Pangenomic and gene ontology analyses in crops consistently find that PAVs are enriched for abiotic stress and disease-response genes [4] , [5] , [9] , [10] , [13] . Increasing evidence has confirmed that PAV is one of the genetic factors underlying variation for agronomic traits such as submergence tolerance (conferred by Sub1A [14] , SNORKEL1 and SNORKEL2 [15] ), phosphous-deficiency tolerance (conferred by Pstol [16] ), anaerobic germination tolerance (conferred by OsTPP7 [17] ), disease resistance (conferred by LRK1 [18] and OsWAK112d [6] ), and plant architecture (conferred by SLB1 and SLB2 [19] ). In addition, fixation of complementary PAVs is believed to contribute to heterosis in hybrid breeding [20] . Asian cultivated rice ( O. sativa L.), which comprises the staple food for half of the global population, was domesticated from common wild rice ( O. rufipogon Griff.) in Asia, and has two subspecies, O. sativa L. ssp. indica and O. sativa L. ssp. japonica (hereafter referred as indica and japonica , respectively) [21] . As two genetically diverged subspecies, indica and japonica varieties display distinct morphological, physiological and biochemical traits, reflecting the adaptive evolution of the two subspecies in divergent natural and human-influenced environments. Various types of post-reproductive barriers exist between indica and japonica rice accessions [22] . Hybrid sterility (HS) is the most commonly found reproductive barrier in indica-japonica crosses, and is often cited as the criterion to classify indica-japonica subspecies [23] . Molecular genetic studies over two decades have revealed three mechanisms of HS in Oryza , which have been designated as the killer-target system, the killer-protector system, and the duplicate gametic lethal system [24] . These involve 9 single-locus HS loci ( Sa [25] , Sc [26] , qHMS7 [27] , S5 [28] , S7 [29] , HSA1 [30] , ESA1 [31] , S1 [32] , [33] , pf12A [34] ) and 3 two-locus HS pairs ( DPL1/DPL2 [35] , S27/S28 [36] , DSG1/DSG2 [37] ). Despite extensive studies of these loci, we still lack efficient methods to fully overcome HS in inter-specific and inter-subspecific hybrid rice, and our understanding of the role of HS in genome evolution remains limited. The yield potential of indica-japonica hybrid rice is estimated to be 15–30% higher than that of the indica intraspecific hybrid rice widely cultivated today. The utilization of strong heterosis in indica-japonica hybrids is one of the most promising future directions in rice breeding [24] , [38] , [39] , [40] , therefore, understanding indica-japonica reproductive isolation is important to unlock their breeding potential. Se/pf12 is a major locus conferring hybrid male sterility in indica-japonica hybrids, which was identified by a large number of studies using different populations [34] , [41] , [42] , [43] , [44] , [45] , [46] , [47] . Artificial disruption of pf12A gene at Se/pf12 locus successfully converts this hybrid sterility locus into a neutral allele [34] . However, the molecular mechanism of pf12A regulating rice HS remains elusive. In this work, we show that a PAV at the Se locus functions as an indica-japonica reproductive barrier by causing HS in indica-japonica crosses. The complementary effect of two adjacent genes at Se locus within the PAV region induces hybrid male sterility (HMS), and thus reproductive isolation between indica and japonica . Evolutionary analyses of Se locus show that the PAV is an important contributor to the postzygotic isolation between the two subspecies, and it also supports the independent domestication of indica and japonica from different O. rufipogon populations. Based on these findings, effective approaches could be designed to break down reproductive barriers in indica-japonica hybrid rice breeding. Identification of Se controlling HMS In order to identify genes responsible for indica-japonica HS, near isogenic lines (NILs) were developed using japonica variety T65 as the recurrent parent and indica variety GLA4 as the donor parent. In the BC 5 F 2 generation, a NIL, E9, was identified that had four substituted segments in the genetic background of T65 (Fig. 1a and Supplementary Fig. 1 ). T65, T65/E9 F 1 hybrids and E9 exhibited similar plant morphology except for anther length (Fig. 1b and Supplementary Figs. 2 and 3a–c ). Pollen staining using both I 2 -KI and TTC showed that male fertility was normal for T65 and E9; however, the T65/E9 F 1 hybrid was semi-sterile, with a mix of fertile and defective pollen (Fig. 1c, d ). Pollen grains of T65 and E9 were larger and spherical (Supplementary Fig. 3d, f–h ), whereas T65/E9 F 1 hybrids produced two kinds of pollen grains: normal, fertile pollen filled with abundant starch granules, and defective pollen filled with cytoplasm but without any starch granules (Supplementary Figs. 3e , i, j and 4a, b ). Defective pollen showed thicker exines and intines than fertile pollen, suggesting that pollen wall formation was also affected in T65/E9 F 1 hybrids (Supplementary Fig. 4c–e ). Semi-thin sections of developing anthers indicated that half of the microspores were aborted in T65/E9 F 1 hybrids starting from the bicellular pollen stage (St11) (Supplementary Fig. 5 ). At the tricellular pollen stage (St12), the aborted pollen resembled St10 vacuolated microspores, whereas normal mature pollen grains were densely stained and filled with starch granules (Supplementary Fig. 5 ). Fig. 1: HMS in T65/E9 F 1 hybrid. a Location of substituted segments on the chromosomes of E9. Chromosomal segments from T65 (white boxes) and GLA4 (black boxes) are indicated. b Morphology of T65, T65/E9 F 1 hybrid and E9 plants. c Pollen stained with I 2 -KI (upper panels) or TTC (lower panels) of T65, T65/E9 F 1 hybrids and E9. Scale bars = 100 μm. Pollen fertility ( d ) and spikelet fertility ( e ) of T65, T65/E9 F 1 hybrids and E9, shown as means ± SD ( n = 10 and 20 biologically independent samples for ( d , e ), respectively). Two-tailed Student’s t tests were performed to determine significant differences (* p < 0.05, ** p < 0.01 and *** p < 0.001). Source data are provided as a Source Data file. 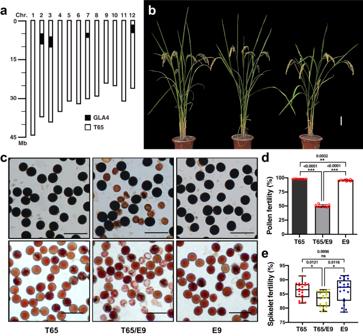Fig. 1: HMS in T65/E9 F1hybrid. aLocation of substituted segments on the chromosomes of E9. Chromosomal segments from T65 (white boxes) and GLA4 (black boxes) are indicated.bMorphology of T65, T65/E9 F1hybrid and E9 plants.cPollen stained with I2-KI (upper panels) or TTC (lower panels) of T65, T65/E9 F1hybrids and E9. Scale bars = 100 μm. Pollen fertility (d) and spikelet fertility (e) of T65, T65/E9 F1hybrids and E9, shown as means ± SD (n= 10 and 20 biologically independent samples for (d,e), respectively). Two-tailed Student’sttests were performed to determine significant differences (*p< 0.05, **p< 0.01 and ***p< 0.001). Source data are provided as a Source Data file. Full size image Segregation analysis of 167 T65/GLA4 BC 5 F 2 plants during E9 construction revealed severely distorted segregation of two SSR markers (RM19 and RM453) on chromosome 12, with significantly lower than the expected 25% homozygous T65 genotype, while SSR markers on chromosome 2, 3 and 7 showed normal 1:2:1 mendelian segregation (Supplementary Table 1 ). 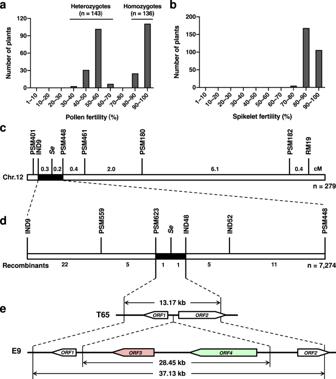Fig. 2: Map-based cloning ofSe. Frequency distribution of pollen fertility (a) and spikelet fertility (b) in the T65/E9 F3segregating population.cSewas preliminarily mapped between IND9 and PSM448 on chromosome 12 using 279 T65/E9 F3plants.dSewas further delimited to a 13.17-kb region between PSM623 and IND48 using 7,274 T65/E9 F4plants.eORFs predicted in the PSM623-IND48 interval. Arrows indicate the orientation ofORFs. Test crosses with T65/E9 F 1 hybrids as the male parent and T65 or E9 as female parents indicated that the male gametes derived from T65 were selectively aborted and T65 alleles were not transmitted to the progeny (Supplementary Table 2 ). Conversely, test cross with T65/E9 F 1 hybrids as the female parent and E9 as the male parent presented 54:74 segregation ratio of T/E and E/E (Supplementary Table 2 ), implying that the female gametes carrying T65 allele is also affected, but at a relatively lower degree compared to male gametes, which is consistent with slightly lower spikelet fertility for T65/E9 F 1 hybrid (Fig. 1e ). For 279 plants of T65/E9 F 3 segregating population, spikelet fertility showed a normal distribution; however, a clear bimodal pattern with an apparent valley at 70–80% was observed for pollen fertility (Fig. 2a, b ). Taking 70–80% as the cut-off region between semi-sterility and fertility, the population segregated for semi-sterility (<70%): fertility (>80%) at the ratio of 1:1 (χ 2 = 0.13 < χ 2 0.05,1 = 3.84), demonstrating monogenic inheritance for the trait. Our results indicated the substituted segment on chromosome 12 contained a gene locus, designated Se as in previous studies [41] , [42] , controlling HMS between T65 and E9, which was closely linked with RM19 and RM453 and appeared to be allelic to several previously identified HMS QTLs [34] , [43] , [44] , [45] , [46] , [47] . Fig. 2: Map-based cloning of Se . Frequency distribution of pollen fertility ( a ) and spikelet fertility ( b ) in the T65/E9 F 3 segregating population. c Se was preliminarily mapped between IND9 and PSM448 on chromosome 12 using 279 T65/E9 F 3 plants. d Se was further delimited to a 13.17-kb region between PSM623 and IND48 using 7,274 T65/E9 F 4 plants. e ORF s predicted in the PSM623-IND48 interval. Arrows indicate the orientation of ORF s. Full size image Complex genomic structural variations at Se locus Linkage analysis of pollen fertility and SSR markers using the above 279 T65/E9 F 3 plants pinpointed the Se locus to an interval between IND9 and PSM448 (Fig. 2c ). Through analysis of 7,274 F 4 plants, Se was further restricted to the genomic region between markers PSM623 and IND48 (Fig. 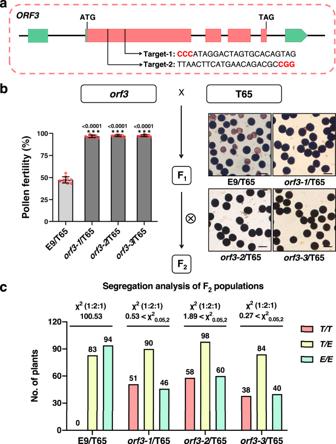Fig. 3: Loss-of-function ofORF3eliminatesSe-mediated HMS and segregation distortion. aPosition of two editing targets inORF3. PAM sequence is highlighted in red.bF1hybrids with threeorf3alleles exhibited normal pollen fertilities. Pollen fertility is shown as means ± SD (n= 10 biologically independent samples). Two-tailed Student’sttests were performed to compare the pollen fertility oforf3/T65 F1hybrids and E9/T65 F1hybrids (***p< 0.001). Scale bars = 50 μm.cSegregation of pollen fertility in F2progeny derived from E9/T65 ororf3/T65 crosses.T/T,E/EandT/Erepresent the homozygous genotype for T65 and E9 and the heterozygous genotype, respectively. Source data are provided as a Source Data file. 2d and Supplementary Table 3 ). Sequence analysis revealed two genes ( ORF1 T65 and ORF2 T65 ) in the 13.17-kb Se region in T65 (Fig. 2e ). ORF1 T65 is predicted to encode a 250-aa protein without any conserved domains and ORF2 T65 is predicted to encode a 466-aa alpha/beta hydrolase family protein. Sequence comparison revealed nucleotide diversity for ORF1 and ORF2 between T65 and E9. Compared with ORF1 E9 , a 378-bp deletion in the last exon and 11 single-nucleotide polymorphisms (SNPs) resulted in a 126-aa deletion and 5 aa substitutions, respectively, in ORF1 T65 (Supplementary Fig. 6 ). Although several indels and SNPs exist between ORF2 T65 and ORF2 E9 , causing premature termination in the predicted ORF2 E9 (Supplementary Fig. 7 ), the major difference in ORF2 is in the promoter region, which is completely different between the two alleles. ORF2 E9 expression could not be detected in anthers or in any other tested tissues (Supplementary Fig. 8 ). In E9, a 28.45-kb insertion was found between ORF1 E9 and the putative ORF2 E9 , containing two additional genes, ORF3 and ORF4 (Fig. 2e ). ORF3 is predicted to encode a 596-aa superfamily II DNA and RNA helicase with a mitochondrial targeting signal (Supplementary Fig. 9 ), and ORF4 is predicted to encode a 523-aa protein with ankyrin repeats (Supplementary Fig. 10 ). ORF3 encodes a sporophytic pollen killer In order to identify the genes responsible for HMS, we used the CRISPR/Cas9 genome editing system to knock out T65 candidate genes in T65 or E9 candidate genes in E9, respectively. Unique target sites were selected in the coding region of each gene to make sure loss-of-function mutations were obtained. Three orf3 homozygous mutants ( orf3-1 to orf3-3 ) and two homozygous mutants each for orf1 T65 , orf2 T65 , orf1 E9 and orf1 T65 orf2 T65 with different editing patterns, respectively, were selected and showed normal pollen viability, suggesting that ORF1 , ORF2 and ORF3 are not essential for the development of male gametophytes (Fig. 3a , Supplementary Fig. 11a–d and Supplementary Tables 4 , 5 ). The mutants were further crossed with T65 or E9 to produce mutant-type Se heterozygotes to test HMS. In contrast to the semi-sterile pollen exhibited by T65/E9 F 1 hybrids and mutant-type F 1 hybrids with orf1 T65 , orf2 T65 , orf1 E9 or orf1 T65 orf2 T65 alleles (Supplementary Fig. 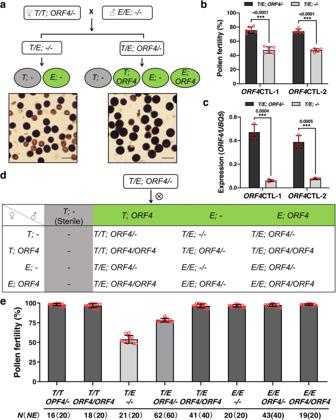Fig. 4:ORF4rescues T65-type pollen in a gametophytic manner. aORF4hemizygous transgenic T0plants were crossed with E9 to generate F1plants without theORF4transgene (T/E; -/-) (left, ~50% pollen fertility) and F1plants with theORF4transgene (T/E;ORF4/-) (right, ~75% pollen fertility). Scale bars = 100 μm.bComparison of pollen fertility between F1plants with (T/E;ORF4/-) and without (T/E;-/-) theORF4transgene. Pollen fertility is shown as means ± SD (n= 6 biologically independent samples).cComparison ofORF4expression between F1plants with (T/E;ORF4/-) and without (T/E;-/-) theORF4transgene. Data are presented as means ± SD (n= 3 biologically independent experiments).dA schematic showing expected genotypes in F2progeny from selfing of F1plants with a single hemizygous copy of theORF4transgene (T/E;ORF4/-).eObserved genotype frequencies and pollen fertility of F2progeny from a selfed F1plant (T/E;ORF4/-). The observed (N) and expected (NE) numbers of individual genotypes among 240 F2progeny are shown. Pollen fertility is shown as means ± SD (n= 10 biologically independent samples). Significant differences were determined by two-tailed Student’sttests (***p< 0.001). Source data are provided as a Source Data file. 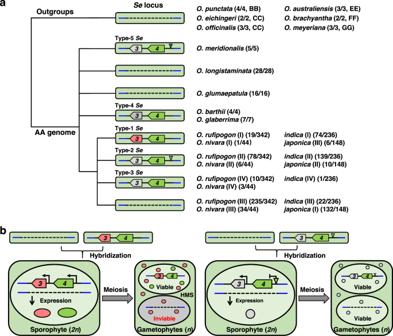Fig. 5: Model for the evolutionary history and genetic action ofSe. aProposal for the evolutionary history ofSelocus. Ancestral wild rice lack the PAV region, andSelocus emerged after the divergence of the AA-genome clade ofOryza. Following the differentiation ofO. meridionalis,O. barthii, andO. rufipogon, theSelocus later evolved in parallel but independent lineages. Based on the haplotype combinations ofORF3andORF4, five main types ofSeloci have been identified.O. rufipogon,O. nivara,indicaandjaponicasamples include four, four, four, and three different types, respectively, and their frequencies are shown next to each type. Full-lengthORF3(red), truncatedORF3(gray),ORF4(green), and deletions inORF4promoter (triangles) are shown.bA proposed model for the molecular genetic basis ofSe-mediated HMS. In hybrids with hemizygous functionalORF3andORF4(left), pollen lacking the PAV region are aborted because of the pollen-killing effect ofORF3and lack of protectiveORF4. When truncated and non-functionalORF3is present (right), only fertile pollen are produced. 11e–h and Supplementary Table 4 ), mutant-type F 1 hybrids with the three orf3 alleles exhibited normal pollen fertility (Fig. 3b ). Moreover, the F 2 families showed the normal 1:2:1 segregation ratio, indicating that loss-of-function of ORF3 restores male fertility in Se heterozygotes and eliminates the segregation distortion (Fig. 3c ). These results are in consistent with normal pollen fertility and 1:2:1 segragation of two heterozygous pf12A (allelic to ORF3 ) mutants [34] . To further study ORF3 ’s function, a genomic fragment containing ORF3 or ORF3 overexpression constructs were introduced into T65. In total, 34 out of 41 (genomic ORF3 ), and 3 out of 28 ( ORF3 overexpression) transgenic lines contained detectable transgenes. Surprisingly, both the transgene-positive lines and transgene-negative lines showed normal pollen fertility (Supplementary Table 6 ). Expression analysis revealed that ORF3 expression in the transgene-positive lines was very low compared with that in T65/E9 F 1 hybrids (Supplementary Fig. 12 ), suggesting that ORF3 is toxic to living cells without ORF4 and its expression should be strictly regulated under T65 genetic background. Direct evidence of ORF3 ’s killing effect was obtained from the transgenic callus experiment in which the selection frequency of Hyg-resistant callus was extremely low for ORF3 compared with the empty vector control (Supplementary Fig. 13a, b ), and transgene-positive calli showed low expression of transgene (Supplementary Fig. 13c ), indicating that the growth of T65 callus was retarded or inhibited when ORF3 was introduced. Similarly, the induction of ORF3 in yeast significantly inhibited the growth of the transformants (Supplementary Fig. 14 ). Our results indicated that ORF3 has a pollen-killing function and acts in a sporophytic manner. Fig. 3: Loss-of-function of ORF3 eliminates Se -mediated HMS and segregation distortion. a Position of two editing targets in ORF3 . PAM sequence is highlighted in red. b F 1 hybrids with three orf3 alleles exhibited normal pollen fertilities. Pollen fertility is shown as means ± SD ( n = 10 biologically independent samples). Two-tailed Student’s t tests were performed to compare the pollen fertility of orf3 /T65 F 1 hybrids and E9/T65 F 1 hybrids (*** p < 0.001). Scale bars = 50 μm. c Segregation of pollen fertility in F 2 progeny derived from E9/T65 or orf3 /T65 crosses. T/T , E/E and T/E represent the homozygous genotype for T65 and E9 and the heterozygous genotype, respectively. Source data are provided as a Source Data file. Full size image ORF4 performs a pollen-protection function in a gametophytic manner The selective abortion of T65-type pollen in T65/E9 F 1 hybrids but not in T65 suggests that a pollen protector is most likely encoded in E9 to eliminate the pollen-killing effect of ORF3 . To test this notion, we transformed intact ORF1 E9 , ORF2 E9 and ORF4 genomic fragments from E9 into T65, respectively. Hemizygous transgenic T 0 plants were further crossed with E9 to produce F 1 hybrids carrying the pollen killer ORF3 (Fig. 4a ). For F 1 plants carrying the ORF4 transgene ( T/E; ORF4 /-), pollen fertility was restored to ~75% (Fig. 4a–c and Supplementary Table 7 ). By contrast, no effect on pollen fertility was observed in the transgene-negative plants ( T/E; -/- ) or F 1 plants with either the ORF1 E9 or ORF2 E9 transgene (Fig. 4b and Supplementary Table 7 ). Moreover, plants in an F 2 population derived from F 1 plants with one hemizygous ORF4 transgene ( T/E; ORF4/- ) segregated as expected (χ 2 = 1.42 < χ 2 0.05,7 = 14.067) (Fig. 4d, e and Supplementary Table 8 ). Se -heterozygotes with homozygous ORF4 ( T/E; ORF4/ORF4 ) were fully fertile, and F 2 plants with genotypes of ( T/T; ORF4/- ) and ( T/T; ORF4/ORF4 ) were recovered (Fig. 4d, e and Supplementary Table 8 ). In contrast, no ( T/T ) plants could be obtained in segregating population derived from T65/E9 F 1 plants (Fig. 3c and Supplementary Table 9 ). These results indicated that ORF4 rescues T65-type pollen in a gametophytic manner. This notion was further supported by the partial restoration of pollen fertility (~75%) in hemizygous T 0 ORF4 overexpression transgenic plants with a T65/E9 genotype (Supplementary Fig. 15 and Supplementary Table 9 ). In addition, we constructed orf4 mutants using the CRISPR/Cas9 genome editing system. Three hemizygous orf4 mutants were obtained, and produced semi-sterile pollen, as expected (Supplementary Fig. 16 and Supplementary Table 10 ). Furthermore, no orf4 homozygous mutant could be recovered in T 1 progeny of these hemizygous orf4 plants (Supplementary Table 11 ). In contrast, orf4 homozygous mutants could be easily obtained when ORF3 was also mutated. As expected, orf3orf4 double mutants with T65/E9 genotypes showed normal pollen fertility (Supplementary Fig. 17 ). Fig. 4: ORF4 rescues T65-type pollen in a gametophytic manner. a ORF4 hemizygous transgenic T 0 plants were crossed with E9 to generate F 1 plants without the ORF4 transgene ( T / E ; -/-) (left, ~50% pollen fertility) and F 1 plants with the ORF4 transgene ( T / E ; ORF4 / - ) (right, ~75% pollen fertility). Scale bars = 100 μm. b Comparison of pollen fertility between F 1 plants with ( T / E ; ORF4 / - ) and without ( T / E ; - / - ) the ORF4 transgene. Pollen fertility is shown as means ± SD ( n = 6 biologically independent samples). c Comparison of ORF4 expression between F 1 plants with ( T / E ; ORF4 / - ) and without ( T / E ; - / - ) the ORF4 transgene. Data are presented as means ± SD ( n = 3 biologically independent experiments). d A schematic showing expected genotypes in F 2 progeny from selfing of F 1 plants with a single hemizygous copy of the ORF4 transgene ( T / E ; ORF4 / - ). e Observed genotype frequencies and pollen fertility of F 2 progeny from a selfed F 1 plant ( T / E ; ORF4 / - ). The observed ( N ) and expected ( NE ) numbers of individual genotypes among 240 F 2 progeny are shown. Pollen fertility is shown as means ± SD ( n = 10 biologically independent samples). Significant differences were determined by two-tailed Student’s t tests (*** p < 0.001). Source data are provided as a Source Data file. Full size image Although both ORF3 and ORF4 localized in cytoplasmic foci (Supplementary Fig. 18 ), no direct interaction of ORF3 and ORF4 was detected using a yeast two-hybrid system (Supplementary Fig. 19 ). qRT-PCR analysis revealed that ORF3 and ORF4 are expressed broadly in different tissues and in all stages of anther development. The expression level in E9 was about twice as high as that in the T65/E9 F 1 hybrids (Supplementary Fig. 20 ), reflecting the different copy numbers (one versus two) in these backgrounds. Evolution of the Se locus To trace the origin of Se locus, we BLAST searched ORF3 and ORF4 homologs in the Genebank database and found that full-length homologs of ORF3 can only be found in Oryza species, indicating it is a gene arose within the Oryza lineage. In contrast, homologs of ORF4 are widely distributed in Poaceae and they all share the conserved protein domain (Supplementary Fig. 21 ), suggesting its conserved function across grasses. To trace the evolutionary history of Se locus in the Oryza genus, we first assayed the presence or absence of the locus by analyzing publicly available high-quality genome sequences of 59 O. sativa [4] , [6] , [48] and 1 O. glaberrima [6] , and PCR amplifying the region spanning part of ORF3 and ORF4 (Supplementary Fig. 22 ) in a large Oryza panel consisting of 787 individuals from 14 Oryza species. Consistent with the BLAST search analysis, target sequences were successfully identified from 363 out of 830 individuals of AA genome, but failed to be amplified from any individuals of GG ( O. meyeriana , 3/3), FF ( O. brachyantha , 2/2), EE ( O. australiensis , 3/3), CC ( O. eichingeri and O. officinalis , 5/5) and BB ( O. punctata , 4/4) karyotypes (Fig. 5a and Supplementary Table 12 ). These results show that the Se locus is polymorphic in the AA rice species, but absent in Oryza species of other karyotypes, suggesting the emergence of the locus is specifically associated with the history of AA-genome Oryza species. Within AA species, the locus can be found in Asian cultivated rice species complex, including O. sativa (230/384), O. nivara (10/44) and O. rufipogon (107/342) and African cultivated rice species complex including O. glaberrima (7/7) and O. barthii (4/4) (Fig. 5a and Supplementary Table 12 ). Surprisingly, it is also present in the basal species of AA genome, O. meridionalis (5/5), but absent in the rest species including O. longistaminata (28/28) and O. glumaepatula (16/16) (Fig. 5a and Supplementary Table 12 ). Further sequence analyses on ORF3 in individuals containing the Se locus identified 14 different haplotypes, among which 13 haplotypes confer truncated form of ORF3 protein, and the haplotype conferring full length protein can only be found in Asian cultivated rice species complex (Supplementary Data 1 ). We tested the effect of truncations by verifying the function of a common truncation form (ORF3 Hap-2 ) and found that its subcellular localization was disrupted (Supplementary Fig. 18 ) and the toxicity effect was abolished in transgenic experiments in yeast and rice callus (Supplementary Figs. 13 , 14 ). These results show that the truncation renders ORF3 Hap-2 non-functional and they also suggest that full-length sequence might be necessary for the ORF3 function, and if so, the functional ORF3 is confined to the Asian cultivated rice species complex, with a significant enrichment of accessions from O. sativa indica subspecies. In contrast, truncated haplotype at ORF4 is extremely rare, which is only found in one indica individual out of 770 accessions assayed in the panel consisting of O. sativa , O. nivara and O. rufipogon (Supplementary Data 2 ). A 369-bp sequence presence/absence variation was identified in the promoter of ORF4 in the panel (Supplementary Data 2 ), and the deletion of the sequence did not affect the subcellular location of ORF4 (Supplementary Fig. 23 ) but significantly reduced the expression level (Supplementary Fig. 24 ), suggesting it is a functional variant in the rice population. A total of 37 haplotypes of the Se locus were identified when ORF3 and ORF4 were considered together, and could be further divided into five Se types according to the function and origins of ORF3 and ORF4 (Fig. 5a and Supplementary Data 3 ). Types 1 to 3 exist in Asian cultivated rice species complex of O. sativa , O. nivara and O. rufipogon , with Type-1 and Type-2 as the two major types representing 27.55% and 64.19% of the rice accessions with the PAV region, respectively (Fig. 5a and Supplementary Tables 13 , 14 ), while Type-4 and Type-5 Se are haplotypes of African cultivated rice species complex and O. meridionalis , respectively (Fig. 5a and Supplementary Tables 13 , 14 ). In sum, our analyses suggest that ORF3 is possibly formed in the Asian rice lineage, and its functional form is maintained in O. sativa indica subspecies in moderate frequency (74/236) (Fig. 5a and Supplementary Tables 13 , 14 ). While in japonica , the majority varieties (132/148) have both ORF3 and ORF4 deleted (Fig. 5a and Supplementary Table 12 ). Therefore, the Se locus is an important isolation barrier between indica and japonica , as it is highly likely to cause hybrid incompatibility when individuals from the two subspecies interbreed. Fig. 5: Model for the evolutionary history and genetic action of Se . a Proposal for the evolutionary history of Se locus. Ancestral wild rice lack the PAV region, and Se locus emerged after the divergence of the AA-genome clade of Oryza . Following the differentiation of O. meridionalis , O. barthii , and O. rufipogon , the Se locus later evolved in parallel but independent lineages. Based on the haplotype combinations of ORF3 and ORF4 , five main types of Se loci have been identified. O. rufipogon , O. nivara , indica and japonica samples include four, four, four, and three different types, respectively, and their frequencies are shown next to each type. Full-length ORF3 (red), truncated ORF3 (gray), ORF4 (green), and deletions in ORF4 promoter (triangles) are shown. b A proposed model for the molecular genetic basis of Se -mediated HMS. In hybrids with hemizygous functional ORF3 and ORF4 (left), pollen lacking the PAV region are aborted because of the pollen-killing effect of ORF3 and lack of protective ORF4 . When truncated and non-functional ORF3 is present (right), only fertile pollen are produced. Full size image PAVs represent a class of SVs that has been suggested to contribute to individual adaptation [49] , [50] . Although PAVs have been mostly linked to roles in ecological and agronomic adaptation in rice [4] , [7] , little is known about possible involvement in speciation. In this study, we identified a PAV contributing to indica-japonica subspecies reproductive isolation through HS. HS maintains the integrity of a species over time, reducing or directly restricting gene flow to or from other species [23] . Consistent with the complex nature of one-locus HS loci identified in previous studies [25] , [26] , [27] , [28] , [29] , [30] , [31] , [32] , [33] , the Se locus in the PAV region studied here comprises two adjacent genes, ORF3 and ORF4 . In hybrids with functional ORF3 and ORF4 , pollen lacking the PAV is aborted. Such pollen lacks protective ORF4 to counteract the pollen-killing effect of ORF3 (Fig. 5b ). Interestingly, ORF3 expression in transgene-positive lines from two independent ORF3 complementation and one overexpression experiments was less than 1/6 of that in T65/E9 F 1 hybrids (Supplementary Fig. 12 ), and no orf4 homozygous CRISPR/Cas9 mutants were obtained in T 0 or T 1 generation (Supplementary Tables 10 , 11 ). These indicate that ORF3 is toxic to living cells without ORF4 , and its expression should be strictly regulated. The toxicity of ORF3 is also supported by the growth inhibition in T65 callus transformed with ORF3 (Supplementary Fig. 13 ) and in yeast cells after ORF3 induction (Supplementary Fig. 14 ). However, one homozygous mutant containing a deletion in pf12B (allelic to ORF4 ) was identified under BL ( pf12 -NJ/NJ) genetic background [34] . One possibility is that this mutant pf12B allele might still preserve some weak function. Genetic verification of this mutant pf12B allele would clarify its functionality. Another possibility is that different copies of ORF4 homologs might exist in BL genetic background, and some ORF4 homologs might be functional, which also needs to be further studied. Consistent with the predicted function of ORF3 as a superfamily II DNA and RNA helicase, ORF3 and ORF4 co-localized in cytoplasmic foci known as Processing bodies (P-bodies) and Stress Granules (SGs) (Supplementary Fig. 18b,e ), which play critical role in mRNA metabolism, including processes such as RNA decay, storage and translation repression [51] , [52] . Plants deficient in P-body components display severe developmental perturbations such as postembryonic lethality and seedling lethality [53] . Correspondingly, transcriptomic analyses revealed that pf12A induced a drastically increased number of differentially expressed genes in the anthers at the mature pollen stage possibly due to aberrant base excision repair and RNA degradation in the gametes [34] . Although the exact role of ORF3 and ORF4 in cytoplasmic foci remained to be further studied, our results showed the ORF3 didn’t affect the formation of P-bodies and SGs (Supplementary Fig. 25 ). In addition to localization in cytoplasmic foci, ORF3 also showed localization in mitochondria (Supplementary Fig. 18g ), suggesting the abortion of pollen might be partially due to impaired mitochondria function and possibly poor energy supply, as shown in male sterilities caused by mitochondria-expressed genes, such as orfH79 , WA352 , S27/S28 and qHMS7-ORF2 [27] , [36] , [54] , [55] . The induction of functional ORF3 in INVSc1 yeast cells significantly inhibited the growth of the transformants, while this growth inhibition was attenuated when ORF3 Δ100 , which encodes ORF3 without mitochondrion localization signal showing disrupted mitochondria localization (Supplementary Fig. 18h ), was transformed (Supplementary Fig. 14 ). In addition, Hyg-resistant secondary calli were apparently propagated from Agrobacterium co-cultivated primary calli transformed with ORF3 Δ100 (Supplementary Fig. 13a, b ). In contrast to low expression of the transgene in ORF3 transgene-positive calli, high expression level of transgenes, although not as high as negative controls, could be obtained in ORF3 Δ100 transgene-positive calli (Supplementary Fig. 13c ), suggesting that the mitochondria and cytoplasmic foci localization of ORF3 are both essential for its function. The PAV is identified between different subspecies of O. sativa which is AA-genome. The outgroups BB-genome O. punctata , CC-genome O. eichingeri , CC-genome O. officinalis , EE-gnome O. australiensis , FF-genome O. brachyantha and GG-genome O. meyeriana lack the PAV region, indicating the absence of PAV is the ancestral condition of the Se locus in Oryza species (Fig. 5a ). The PAV is only found in AA genome of Oryza species, and remains polymorphic across different species in Asian and African cultivated rice species complexes, surprisingly, it is also found in basal species of AA genome O. meridionalis but not in other AA species including O. glumaepatula and O. longistaminata . This pattern could have been caused by recent gene introgression at the Se locus across different species or independent loss of the Se locus in O. glumaepatula and O. longistaminata . These results clearly show that the locus was formed within the AA genome species of Oryza genus, and particularly, ORF3 is only found within Asian cultivated rice species complex. Monophyletic origin [56] , polyphyletic origin [7] , [57] , and japonica -to- indica introgression theories [58] have been advanced to explain the origin and domestication of Asian cultivated rice. We found 89.19% japonica ( japonica (I)) lack the PAV and 90.68% indica ( indica (I), indica (II) and indica (IV)) contain the PAV (Fig. 5a and Supplementary Table 12 ). Moreover, the PAV is also segregating in the population of O. rufipogon , the presumed wild progenitor of domesticated rice. These patterns are consistent with the scenario that japonica and indica originated from different O. rufipogon populations respectively and showed different haplotype distributions at the locus as a result. Therefore, the haplotype diversity pattern at the Se locus is consistent with polyphyletic origin and independent domestication of indica and janopica from different ancestral O. rufipogon populations. In indica (II)/ japonica (I) F 1 hybrids, no gametes were selectively aborted through Se function due to the lack of pollen killer ORF3 , generating minor types such as indica (III) (9.32% indica ) and japonica (II) (6.76% japonica ) (Fig. 5 ). Through repetitive backcrosses of indica (I) with japonica (I) during artificial selection, the rare japonica (III) (4.05% japonica ) could also be created (Fig. 5a ). For example, pedigree analyses indicated that japonica (III) varieties WYG7 and LG31 were bred through repeatedly backcrossing indica varieties derived from IR54 or TDK with different japonica varieties (Supplementary Fig. 26 ). Our results demonstrate that the differentiation of two subspecies of O. sativa L. can be partially reversed through artificial selection, which is consistent with the genetic mixture of indica and japonica shown in the evolutionary study of S5 [59] . Despite clear examples of PAV controlling agronomic traits in different species, PAV events have been proposed to be largely restricted to genes with signatures of reduced essentiality, so called dispensable genes, and are recent additions to plant genomes [60] . Our study presents a PAV contributing to reproductive isolation of the two subspecies of Asian cultivated rice. Although the origin and maintenance mechanisms of the PAV remain unclear for the moment, the near fixation of the PAV in indica suggests it might be favorable in environment adaptation and/or human selection during the indica domestication process. Future study of ORF3 and ORF4 in response to different environmental cues may help to elucidate its beneficial effects in adaptation. Reproductive isolation hinders the utilization of strong hybrid vigor in indica-japonica crosses in rice. Besides major effect on HMS, Se was also found to affect female gamete development at a lower degree (Supplementary Table 2 and Fig. 1e ), which is consistent with result of pf12A [34] . Therefore, Se is one of the most important target to overcome indica-japonica HS. In our study, Type-3 Se allele with non-functional ORF3 and full-length ORF4 was identified as a neutral haplotype in O. rufipogon (IV), O. nivara (IV) and indica (IV) (Fig. 5a and Supplementary Data 3 ), and could be crossed into current varieties to build natural hybrid-compatible lines. Alternatively, a neutral Se allele could be artificially generated by disrupting ORF3 using CRISPR/Cas9 knockout or base editing strategies. Through genetic modification of Se and other indica-japonica hybrid sterility loci such as S5 , Sa and Sc , widely-compatible lines could be created to break down reproductive barriers in indica-japonica hybrid rice breeding, thus having important implications in agriculture. Plant materials and growth conditions O. sativa ssp. japonica T65, NIL E9 and T65/E9 F 1 hybrid were used in gene cloning and functional analysis. The wild and cultivated rice species used for haplotype investigation and evolutionary analysis came from our laboratory or were provided by the International Rice Research Institute (Los Baños, Philippines), Guangxi Academy of Agricultural Sciences (Guangxi, China) and Yunnan Academy of Agricultural Sciences (Yunnan, China). All plant materials were grown at the experimental farm of South China Agricultural University, Guangzhou, China. Phenotypic characterization To analyze pollen fertility, panicles at the flowering stage were fixed in FAA fixative [89% (v/v) ethanol, 6% (v/v) formaldehyde and 5% (v/v) acetic acid], and more than 200 pollen grains stained with 1% potassium iodide (I 2 -KI) solution were observed with an optical microscope (BK6000, OPTEC, China) to obtain pollen phenotype. To assess pollen vitality, pollen grains at the anthesis stage were collected and stained with 0.1% 2,3,5-triphenyl-2h-tetrazolium chloride (TTC) solution for 30 min before microscopic examination. A stereo microscope (SZ810, OPTEC, China) was used to observe the spikelets and anthers. Spikelet fertility was measured as the seed-setting rate of 20 individual main panicles. Cytological analysis For scanning electron microscopy (SEM) and transmission electron microscopy (TEM) observations, mature anthers of T65, E9 and T65/E9 F 1 hybrid were pre-fixed in 0.1 M sodium phosphate buffer containing 4% glutaraldehyde (pH7.0) at 4 °C overnight. For SEM, pre-fixed samples were rinsed 3 times with 0.1 M phosphate buffer (pH7.0), and then were post-fixed for 2 h with 1.5% osmium tetroxide (OsO 4 ) in PBS (pH7.0). After rinsing with PBS (pH7.0) and ethanol dehydration (30% to 100%), samples were exchanged 3 times with isoamyl acetate. Then, the fixed samples were dried with a critical point drier and coated with gold. The anther and pollen grains were observed using a scanning electron microscope (EVO MA 15, ZEISS, Germany) with an acceleration voltage of 10 kV. For TEM, pre-fixed samples were rinsed 3 times with PBS (pH7.0), post-fixed with 1.5% OsO 4 in PBS (pH7.0) for 2 hours, and rinsed again 3 times with PBS (pH7.0). The post-fixed anthers were subjected to ethanol dehydration (30% to 100%) and transferred gradually to 100% resin. Super-thin sections (60 nm) were collected on uncoated nickel grids, and double stained with uranyl acetate and citrate aqueous solution as described previously [61] . Images were obtained with a transmission electron microscope (Talos L120C, FEI, America) operated at 80 kV. To observe the development of anther and pollen, anthers at different stages were pre-fixed in FAA fixative, and were then embedded using Technovit Embedding Kits (Technovit 7100, Germany). Semi-thin sections (2 μm) were prepared using a microtome (RM2235, Leica, Germany), followed by staining with 0.5% toluidine blue. The stained sections were imaged with an optical microscope (BK6000, OPTEC, China). Fine mapping of Se locus and sequence analysis A mapping population was generated from a cross between T65 and E9. Two hundred and seventy-nine plants from the F 3 population were used to analyze the linkage between pollen fertility and SSR markers for primary gene mapping. Additional SSR and InDel markers were designed in the IND9-PSM448 interval based on the polymorphisms between japonica Nipponbare and indica 9311. Fine mapping was performed using 7274 plants from the F 4 population, and the final region was further confirmed through genotypic segregation and phenotypic analysis of the progeny of key recombinants. The genomic DNA sequence of Se region was amplified from T65 and E9 using KOD-Plus-Neo DNA polymerase (TOYOBO, Japan) and assembled using SnapGene. All primers are listed in Supplementary Data 4 . Full-length cDNA cloning and qRT-PCR analysis Total RNA from young panicles of T65 and E9 were extracted using TRIZOL reagent (Invitrogen, America) according to the manufacturer’s instructions. First-strand cDNA was reverse transcribed using a Hifair® III 1st Strand cDNA Synthesis Kit (YEASEN, China). The predicted coding regions of candidate genes were amplified from cDNA and sequenced. RACE assay was performed by nested PCR with the SMARTer RACE cDNA Amplification kit (Clontech, America) following the manufacturer’s instructions. The anthers in different stages (meiocyte stage, microspore stage, early-bicellular stage, late-bicellular stage, and tricellular stage) from T65, E9 and T65/E9 F 1 hybrids, along with different tissues of E9 were selected for qRT-PCR assays according to a previous study [62] , and the expression values were normalized to UBQ5 transcript levels. Constructs for rice transformation For complementation analysis, four genomic fragments (7,641-bp, 8,082-bp, 8,463-bp and 10,755-bp) were amplified from E9 and cloned into the binary vector pCAMBIA1300 to obtain the ORF1 E9 CTL, ORF2 E9 CTL, ORF3 CTL, and ORF4 CTL constructs. All constructs were introduced into T65 using Agrobacterium -mediated transformation. Transformation of ORF3 CTL was conducted twice in independent experiments, and 34 transgene-positive lines were obtained in total. Mutations of Se were constructed using the CRISPR/Cas9 vector system as previously reported [63] , and target sites were designed by the web-based tool CRISPR-GE/targetDesign ( http://skl.scau.edu.cn/ ) [64] . Constructs of orf1 T65 , orf2 T65 and orf1 T65 orf2 T65 were introduced into T65; orf1 E9 and orf3 constructs were transformed into E9; and orf3orf4 was introduced into T65/E9 F 1 hybrids. For generation of orf4 mutants, constructs of three orf4 with different target sites in the coding region of ORF4 (target-1: CCGAAGATTACGAATCTTGGACA; target-2: CATATCTCTCACTTCGCGTATGG; target-3: TGTTCGCCGATGCGCCGTAACGG) were transformed into E9 or T65/E9 F 1 hybrids in four independent experiments (Supplementary Table 10 ), and two types of frameshift mutations in three independent hemizygous orf4 mutants were obtained. Because we didn’t detect ORF2 E9 expression in the tested materials (Supplementary Fig. 8 ), we didn’t construct CRISPR/Cas9 vector targeting ORF2 E9 to generate orf2 E9 . Overexpression constructs ( ORF3 OE and ORF4 OE), in which coding sequence of E9 was driven by CaMV 35 S promoter, were transformed into T65 and T65/E9 F 1 hybrids, respectively, to verify the killer function of ORF3 and the protector function of ORF4 , respectively. Rice transformations were performed by Edgene Biotechnology Co., Ltd. Wuhan, China. For pollen sterility analysis and qRT-PCR analysis of single given T 0 transgenic plant, standard deviation was calculated from the 3 plants generated from a single positive callus. Three or more independent T 0 transgenic plants were used as biological replicates. Agrobacterium -mediated callus transformation Overexpression constructs of eGFP (empty vector), ORF3-eGFP , ORF3 Δ100 - eGFP (with 5’ sequence encoding N-terminal 100-aa of ORF3 deleted), ORF3 HJX74 - eGFP ( ORF3 Hap-2 - eGFP ) were transferred into Agrobacterium tumefaciens strain EHA105. Sterilized mature seeds were inoculated on UINB medium and cultured at 28 °C in the dark. After 7 days of incubating, the calli were collected and used for transformation. After 3 days of cocultivation with Agrobacterium at 25 °C in constant darkness on N6D-Acetosyringone (AS) medium (30 g/L sucrose, 10 g/L glucose, 0.3 g/L casamino acids, 4.39 g/L N6D medium salt mixture, 2.878 g/L L-proline, and 2.8 mg/L 2,4-D, 20 mg/L AS, pH 5.4), the calli were washed two or three times with sterile water and rinsed once with sterile water containing 500 mg/L carbenicillin. Then, the calli were cultured on UINB medium containing 50 mg/L hygromycin B (Hyg, Merck), 400 mg/L carbenicillin for 30 days at 32 °C in constant light. Selection frequency of Hyg-resistant callus represents data from 3 groups of independent experiments, with ~50 transformed calli per group. Six (for ORF3-eGFP ) and more than ten (for others) Hyg-resistant calli were used to test the expression of transgenes. Susceptibility assay with inducible ORF3 expression S. cerevisiae INVSc1 transformed with a vector harboring coding sequence of ORF3 gene from E9 (pYES2- ORF3 and pYES2- ORF3 Δ100 ), HJX74 (pYES2- ORF3 HJX74 ) or empty vector (pYES2-CT) was pre-cultured overnight at 30 °C in SC-Ura liquid medium (Coolaber, China) containing 2% glucose (SCGlu-Ura medium). To induce the ORF3 gene driven by GAL1 promoter, the transformant was inoculated at an initial concentration equivalent to OD600 = 0.1 into 50 mL of SC-Ura containing 3% galactose and 2% raffinose (SCGal-Ura medium), and cultured for 92 h at 30 °C. The growth of yeast cells was monitored by OD600. In the case of the reference experiment without induction of the ORF3 gene expression, SCGal-Ura medium was replaced with SCGlu-Ura medium, and the culture time is 40 h. Subcellular localization of ORF3 and ORF4 For subcellular localization, the ORF3 and ORF4 coding region (minus the stop codon) were cloned into the pRTVcGFP vector, and plasmids were prepared using the FinePure EndoFree Plasmid Mini Kit (GENFINE, China). Constructs of eGFP (empty vector), ORF3-eGFP , ORF3 Δ100 - eGFP , ORF3 HJX74 - eGFP , ORF4-eGFP ( ORF4 Hap-1 - eGFP ), ORF4 Hap-2 - eGFP , ORF4 Hap-3 - eGFP and ORF4 Hap-12 - eGFP were transformed or co-transformed with plasmid encoding the cytoplasmic foci marker AtTZF1-mCherry [65] into rice protoplasts using the polyethylene glycol method. Following incubation for 14 to 20 h at 28 °C, fluorescence was observed using confocal microscopy (TCS SP8, Leica, Germany). Transformed protoplasts were stained with mitochondrion-specific dye MitoTracker Deep Red (Invitrogen, America) to view mitochondira signal. Phylogenetic and evolutionary analysis of Se locus To identify putative homologs of ORF3 and ORF4, full-length protein sequences were used to query the NCBI database ( https://www.ncbi.nlm.nih.gov/ ). Sequence alignment and neighbor-joining phylogenetic tree construction were performed using MEGA7 software (bootstrap replication = 1000). To trace the evolutionary history of the Se locus, genomic DNA was extracted from 787 rice samples, including 4 O. punctata , 2 O. eichingeri , 3 O. officinalis , 3 O. australiensis , 2 O. brachyantha , 3 O. meyeriana , 28 O. longistaminata , 16 O. glumaepatula , 5 O. meridionalis , 4 O. barthii , 342 O. rufipogon , 44 O. nivara , 6 O. glaberrima , and 325 landraces (consisting of 217 indica and 108 japonica ) from Rice Diversity Panel 2 [66] . For all materials that contained the PAV region, ORF3 and ORF4 were sequenced and assembled using SnapGene. All of the sequences obtained and an additional 60 publicly available high-quality genome sequences [4] , [6] , [48] were used for haplotype investigation and evolutionary analysis. All rice materials are listed in Supplementary Data 5 . Reporting summary Further information on research design is available in the Nature Portfolio Reporting Summary linked to this article.